Ferroelectric tunnel junctions for information storage and processing Ferroelectric random access memories (FeRAMs), in which information is encoded through the ferroelectric polarization, are commercially available products with fast write speed, large read/write cycle endurance and low-power consumption [1] . In these ferroelectric capacitors, a ferroelectric thin film (typically 100 nm thick) is sandwiched between two electrodes and the remnant polarization is switched by applying an electric field between the electrodes. The widespread development of these memories is however limited owing to the capacitive readout of the information (the polarization) that prevents the scalability of FeRAMs up to gigabit densities and necessitates the rewriting of information after readout (destructive readout) [2] . In ferroelectric diodes, the current across a thick ferroelectric can be modulated by the polarization at the ferroelectric/electrode interface, giving rise to a non-destructive, resistive readout of the information [3] , [4] . But in these devices, the large thickness of the ferroelectric layer results in very low readout currents, limiting their miniaturization. As the ferroelectric layer thickness is decreased to a few nanometres, electronic conduction is greatly enhanced as quantum-mechanical tunnelling through the ferroelectric becomes possible [5] , [6] . These devices in which two electrodes sandwich a ferroelectric tunnel barrier are called ferroelectric tunnel junctions (FTJs). The tunnel transmission may be strongly modulated by the ferroelectric polarization producing giant tunnel electroresistance (TER) with OFF/ON resistance ratios reaching 10 4 (refs 7 , 8 ). Moreover, the readout current densities are much larger than in ferroelectric diodes, thereby opening the path to possible applications as high-density ferroelectric memories with non-destructive readout. Here we review the fast progress of the nascent field of FTJs and give perspectives for new physical effects and future applications. We first summarize possible electron transport mechanisms that occur when voltage is applied across ultrathin films of ferroelectrics. We then focus on experimental reports that evidence a direct correlation between ferroelectric switching and resistive switching, from local probes experiments on ferroelectric surfaces to solid-state devices. Various approaches such as strain or electrode/barrier interface engineering have been introduced, resulting in a large increase of the OFF/ON resistance ratio. The key features of state-of-the-art FTJs are then described in terms of potential applications as non-volatile memories. This careful crafting of the structural and electronic details of the junction not only yields better performing devices, but also brings additional functionalities. One degree of freedom to engineer the response of these junctions is the domain structure in the ferroelectric barrier. It was recently used to achieve a new form of memristive behaviour, expanding the scope of applications of ferroelectric junctions from digital information storage to brain-inspired computation. In addition, ferroelectric switching in the barrier can induce modifications of the magnetic properties when using ferromagnetic electrodes, or phase transitions in strongly correlated oxides. This functionality also opens new routes for the nanoscale control of their electronic and spintronic response. In this section, we review the influence of ferroelectric polarization ( P ) on the transport properties of an ultrathin ferroelectric layer sandwiched between two metallic electrodes. The imperfect screening of polarization charges at the interface results in a distorted potential profile whose asymmetry and average height can depend on the polarization direction, see Box 1 . This is the main mechanism producing TER in FTJs. Although this review mainly deals with FTJs, direct tunnelling is not the only possible electronic transport mechanism across ultrathin ferroelectric films. Pantel and Alexe [9] calculated the influence of polarization charge effects on the current flowing through ultrathin ferroelectrics (in the limit of fully depleted ferroelectrics) within three possible transport mechanisms: direct tunnelling, Fowler–Nordheim tunnelling and thermionic emission ( Fig. 1a ). 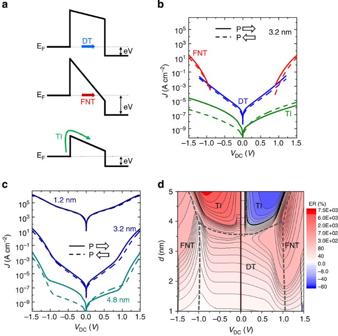Figure 1: Electron transport across ultrathin ferroelectrics. (a) Illustration of three possible transport mechanisms through ultrathin ferroelectrics: direct tunnelling (DT), Fowler–Nordheim tunnelling (FNT) and thermionic emission (TI). (b) Current densities (J) versus voltage (VDC) of the contributions from DT, FNT and TI through a 3.2-nm-thick ferroelectric. (c) Total current densitiesJ=JDT+JFNT+JTIversusVDCfor a 1.2-, 3.2- and 4.8-nm-thick ferroelectric. Inbandc, solid and dashed lines stand forPright andPleft, respectively. (d) Corresponding electroresistance (ER) as a function of voltage anddas the ferroelectric thickness. The dashed lines illustrate the boundaries where each DT, FNT and TI mechanism dominates. The parameters used inb–dareP=3 μC cm−2,εstat=60,εifl=10, m*=1, A**=106Am−2K−2,λ1=0.08 nm,λ2=0.055 nm,ε1=8,ε2=2, Φ1,2=1. ((b–d) adapted, with permission from ref.9, copyright 2010 by The American Physical Society.) Figure 1b illustrates the contribution of each transport mechanism for an intermediate barrier thickness: direct tunnelling current is prominent at low voltage and Fowler–Nordheim tunnelling dominates at large voltage. As the barrier thickness increases, the direct tunnelling current decreases exponentially and the current due to thermionic emission dominates ( Fig. 1c ). Interestingly, the electroresistance (ER; defined here as (J P→ −J P← )/J P← ) increases in the low bias regime ( V DC =−0.1 V) as the barrier thickness increases [9] , [10] ( Fig. 1d ). For large thicknesses, when transport is dominated by thermionic injection, the ER reaches high values and its sign reverses at positive voltage. Nevertheless, the large increase of the ER in the thermionic injection regime is at the expense of a strong decrease of the read current ( Fig. 1c ) [9] . Figure 1: Electron transport across ultrathin ferroelectrics. ( a ) Illustration of three possible transport mechanisms through ultrathin ferroelectrics: direct tunnelling (DT), Fowler–Nordheim tunnelling (FNT) and thermionic emission (TI). ( b ) Current densities ( J ) versus voltage ( V DC ) of the contributions from DT, FNT and TI through a 3.2-nm-thick ferroelectric. ( c ) Total current densities J = J DT + J FNT + J TI versus V DC for a 1.2-, 3.2- and 4.8-nm-thick ferroelectric. In b and c , solid and dashed lines stand for P right and P left, respectively. ( d ) Corresponding electroresistance (ER) as a function of voltage and d as the ferroelectric thickness. The dashed lines illustrate the boundaries where each DT, FNT and TI mechanism dominates. The parameters used in b – d are P =3 μC cm −2 , ε stat =60, ε ifl =10, m*=1, A**=10 6 Am −2 K −2 , λ 1 =0.08 nm, λ 2 =0.055 nm, ε 1 =8, ε 2 =2, Φ 1,2 =1. (( b – d ) adapted, with permission from ref. 9 , copyright 2010 by The American Physical Society.) Full size image Experimentally, the frontier between these different transport mechanisms is hard to draw as it depends on various specific parameters (dielectric constants, screening lengths, interface barrier heights and effective mass). Nevertheless, specific signatures of each transport mechanism can be identified through voltage and temperature dependences of the electronic current. For example, thermionic emission is a thermally activated process that should in principle lead to strong variations with temperature; this is not the case for direct tunnelling. The interplay between electronic transport and ferroelectricity is in reality much more complex than what can be inferred from classical electrostatic models based on polarization charge effects. As ferroelectrics are all piezoelectric, converse piezoelectric effects result in a modification of the ferroelectric thickness when a voltage is applied. The voltage dependence of this modulation is reversed when the ferroelectric polarization is switched. This influences the current across a ferroelectric when read at a large voltage [11] . However, FTJs are usually read at low voltage to avoid destabilizing the ferroelectric state, and the piezoelectric coefficient may be limited in clamped ultrathin films [12] , [13] . In-depth investigations on model systems have been performed by ab initio calculations for direct tunnelling transport. The tunnel current is dependent on the product of interface transmission functions and on the decay rate of the evanescent states within the barrier (related to its complex band structure) [14] . In the case of Pt/BaTiO 3 /Pt tunnel junctions, the modifications of the electronic structure related to ferroelectric displacements strongly influence the transmission of the tunnel barrier via a modulation of the complex band structure of the barrier [15] . The interface transmission probability at the Pt/BaTiO 3 interface varies with the orientation of the polarization [15] . For SrRuO 3 /BaTiO 3 /SrRuO 3 junctions, asymmetries in the interface terminations (BaO/RuO 2 and TiO 2 /SrO) induce an asymmetry of the amplitude of the ferroelectric displacements when the polarization points towards one or the other interface. As a result, a change of the band gap of BaTiO 3 for the two orientations of the polarization modifies the tunnelling decay rate in BaTiO 3 , which leads to a change in the tunnel current [16] . Box 1: A simplified picture of ferroelectric tunnel barriers. At the surface of a ferroelectric, polarization charges are usually present and, depending on their sign, will repel or attract electrons. This occurs over a short distance in the electrode beyond which the density of electrons resumes its normal value: the electrons near the interface screen the polarization charges. In Thomas–Fermi theory, the screening length is a function of the electronic density of states at the Fermi level. For very good metals, the Thomas–Fermi screening length can be shorter than a tenth of nanometre. For semiconductors, it can reach tens of nanometres and screening is imperfect. However, as emphasized by Stengel et al. [97] , the actual effective screening length differs from the one defined by Thomas–Fermi and strongly depends on the microscopic properties of the ferroelectric/electrode interface system. This incomplete screening gives rise to an additional electrostatic potential at the ferroelectric/electrode interface (>0 when P points to the interface and <0 when P points away from the interface). We now consider an ultrathin ferroelectric layer sandwiched between two different electrodes with more efficient screening on the left side than on the right side (Figure Box 1). The larger the screening length over the dielectric constant of the electrode, the larger is the additional electrostatic potential at the electrode/ferroelectric interface. For simplicity, we suppose that the initial electronic potential barrier is rectangular (that is, identical barrier heights for the left and right interfaces). Polarization charge effects induce an asymmetric modulation of the electronic potential profile [10] , [11] . When P is reversed, the asymmetry of the electronic potential profile is reversed. This results in the barrier height being in average higher when P points to the left than when P points to the right. Because the tunnel transmission depends exponentially on the square root of the barrier height, the junction resistance will depend on the direction of P . The asymmetry between the two ferroelectric/electrode interfaces is thus essential to modulate the current transmission of the ferroelectric barrier. The use of different electrode materials is, however, not mandatory and the asymmetry may come from the interfaces only because of different interface terminations [16] , an ultrathin dielectric layer at one of the interfaces [98] or pinned interface dipoles [99] , [100] . The figure depicts the polarization-induced variation of the tunnel barrier height in FTJs and the potential profile across the metal 1 (M1)/ferroelectric/metal 2 (M2) heterostructure for two orientations (right and left) of the ferroelectric polarization ( P ). The ferroelectric is thin enough to be fully carrier depleted, and charges of the ferroelectric are more efficiently screened in M1 than in M2 ( λ 1 / ε 1 < λ 2 / ε 2 , λ i stands for the screening length and ε i the dielectric constant, i=1 and 2). Owing to electrostatic effects, the average barrier height is small (Φ − ) or large (Φ + ), when P points to the right or to the left, respectively. The concept of FTJs was proposed by Esaki in 1971 (ref. 17 ). It was forgotten for about 30 years as ferroelectricity was believed to vanish at critical thicknesses well above the nanometre range [18] . Owing to tremendous improvements in the growth of high-quality ferroelectric films and in the characterization techniques of ferroelectricity, ultrathin films of ferroelectric materials were experimentally demonstrated in the early 2000s (refs 19 , 20 , 21 , 22 , 23 , 24 , 25 , 26 , 27 ). First experiments performed in Jülich resulted in the demonstration of resistive switching of 400% at room temperature in junctions based on ultrathin films of PbZr 0.52 Ti 0.48 O 3 sandwiched between SrRuO 3 and Pt [28] . A few years later, the same group proposed a method to ascribe resistive switching to ferroelectric switching in ferroelectric capacitors, and concluded that their initial results were probably not related to ferroelectricity [29] . Combining local-probe techniques based on atomic force microscopy (AFM), three groups unambiguously demonstrated, in 2009, the correlation between ferroelectricity and resistive switching on bare surfaces of ferroelectrics [30] , [31] , [32] . Highly strained ultrathin films of BaTiO 3 show large TER, of up to 750 for 3-nm-thick films, correlated with ferroelectricity by combining images of ferroelectric domains by piezoresponse force microscopy (PFM) and resistance maps of the domains with conductive-AFM (C-AFM) [30] . Similar results were independently observed through ultrathin films of BaTiO 3 by Gruverman et al. [32] with additional local current versus voltage ( I versus V DC ) curves that were fitted by direct tunnelling models. Maksymovych et al. [31] locally connected a surface of PbZr 0.2 Ti 0.8 O 3 (30 nm) with a C-AFM tip; they collected the local DC piezoresponse of the ferroelectric and measured simultaneously the current as a function of the voltage applied through the ferroelectric. A large change of current was directly correlated to ferroelectric switching. This 500-fold current contrast at large negative voltage was described within the Fowler–Nordheim tunnelling regime ( Fig. 2a ) [31] . We note that, for such a thick barrier of PbZr 0.2 Ti 0.8 O 3 , Fowler–Nordheim tunnelling involves electron transport in the ferroelectric itself that may occur via hopping or other mechanisms, although the Schottky barrier resistance seems to be predominant. 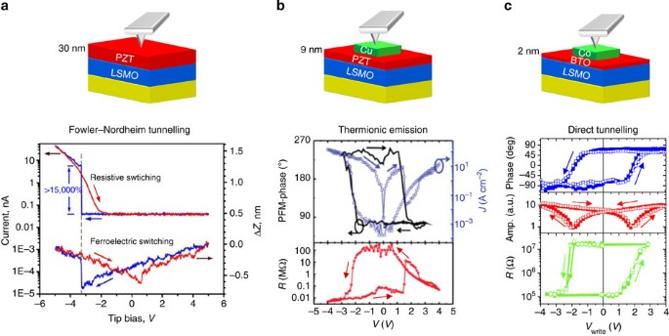Figure 2: Ferroelectric polarization control of resistive switching. (a) Simultaneous measurements of local conductance (current versus tip bias) and piezoresponse on the surface of a 30-nm PZT film (adapted from ref.31, with permission from AAAS). (b) Current density versus voltage and remnant PFM phase hysteresis on the same Cu/PZT/LSMO device (thickness: 9 nm; area: 0.6 μm2) in consecutive measurements. The lower panel provides resistanceRversus voltage (reprinted, with permission from ref.36, copyright 2011 American Chemical Society). (c) Out-of-plane PFM phase (blue) and amplitude (red) measurements on a typical Au/Co/BTO/LSMO ferroelectric tunnel junction (diameter of 500 nm). Resistance (in green) versus voltage pulse height (Vwrite) for a similar capacitor measured in remanence (Vread=100 mV) after applying successive voltage pulses of 100 μs. Open and filled circles represent two different scans to show reproducibility (adapted from ref.37). Each device and its measurement configuration with the AFM tip are sketched in the top panels. PZT, LSMO and BTO stand for PbZr0.2Ti0.8O3, La0.7Sr0.3MnO3and BaTiO3, respectively. Figure 2: Ferroelectric polarization control of resistive switching. ( a ) Simultaneous measurements of local conductance (current versus tip bias) and piezoresponse on the surface of a 30-nm PZT film (adapted from ref. 31 , with permission from AAAS). ( b ) Current density versus voltage and remnant PFM phase hysteresis on the same Cu/PZT/LSMO device (thickness: 9 nm; area: 0.6 μm 2 ) in consecutive measurements. The lower panel provides resistance R versus voltage (reprinted, with permission from ref. 36 , copyright 2011 American Chemical Society). ( c ) Out-of-plane PFM phase (blue) and amplitude (red) measurements on a typical Au/Co/BTO/LSMO ferroelectric tunnel junction (diameter of 500 nm). Resistance (in green) versus voltage pulse height ( V write ) for a similar capacitor measured in remanence ( V read =100 mV) after applying successive voltage pulses of 100 μs. Open and filled circles represent two different scans to show reproducibility (adapted from ref. 37 ). Each device and its measurement configuration with the AFM tip are sketched in the top panels. PZT, LSMO and BTO stand for PbZr 0.2 Ti 0.8 O 3 , La 0.7 Sr 0.3 MnO 3 and BaTiO 3 , respectively. Full size image These and other demonstrations of ferroelectricity-induced ER on bare surfaces of ferroelectrics using local probes [30] , [31] , [32] , [33] , [34] , [35] then triggered the development of solid-state resistive devices based on ferroelectrics. In 2011, Pantel et al. [36] fabricated submicron devices based on an ultrathin film of PbZr 0.2 Ti 0.8 O 3 of 9 nm sandwiched between a bottom electrode of La 0.7 Sr 0.3 MnO 3 and a top one of Cu. They observed the correspondence between ferroelectricity, via PFM versus voltage loops acquired through the top Cu electrode, and the ER measured by I versus V DC ( Fig. 2b ). An OFF/ON ratio of 1,500 was found, with a relatively high current of 10 A cm −2 at low read voltage in the ON state. The transport properties were described by the thermionic emission mechanism [36] . In 2012, Chanthbouala et al. [37] designed tunnel junctions based on highly strained 2-nm-thick BaTiO 3 films grown on La 0.7 Sr 0.3 MnO 3 bottom electrodes with arrays of submicron Au/Co top electrodes. Local PFM phase and amplitude versus voltage hysteresis were observed through the top electrode, indicating that the BaTiO 3 is ferroelectric inside the device ( Fig. 2c ). The remnant resistance of the device was shown to change hysteretically with OFF/ON ratios of 100 after applying voltage pulses of 100 μs with coercive fields matching ferroelectric switching events detected by PFM [37] . Over recent years, solid-state FTJs with various ferroelectrics such as BaTiO 3 (refs 8 , 37 , 38 , 39 , 40 , 41 , 42 ), PbZr 0.2 Ti 0.8 O 3 (ref. 43 ) and BiFeO 3 (refs 7 , 44 ) have been demonstrated by several groups (information can be found in Table 1 ). Performance metrics such as OFF/ON ratios, write energies, data retention, scalability and endurance are critical to consider potential applications of FTJs as non-volatile memories. Table 1 Survey of experimental reports of tunnel electroresistance with ferroelectric tunnel junctions. Full size table Previously mentioned Co/BaTiO 3 /La 0.7 Sr 0.3 MnO 3 tunnel junctions ( Fig. 2c ) showed large OFF/ON ratios (100) with good reproducibility and low write current densities (10 4 A cm −2 ), as the driving force for resistive switching is the electric field [37] . The ON and OFF states can be written with single-voltage pulses down to 10 ns, suggesting high speed with low write energy. The transport properties were investigated with I versus V DC in the ON and OFF states, and at low DC voltage. They showed non-linear characteristics and a weak temperature dependence, indicating that electron transport occurs mainly in the direct tunnelling regime [45] . In order to gain further insight into the physical mechanisms that induce TER, I versus V DC can in principle be fitted with classical tunnelling models [32] , [45] . There are, however, too many unknown physical parameters (dielectric constant, polarization, effective screening lengths, effective mass of tunnelling electrons and so on) to reasonably fit experimental data. To overcome this limitation, Zenkevich et al. [41] performed hard X-ray photoemission experiments to gather more information on the electrode/ferroelectric interfacial electronic properties. They successively determined the interfacial BaTiO 3 /Pt and Cr/BaTiO 3 barrier heights, and used these parameters to fit I versus V DC measured on Cr/BaTiO 3 /Pt tunnel junctions in the ON and OFF states at room temperature. Hence, the OFF/ON ratio of 30 at room temperature in these FTJs can be interpreted by a modulation of the potential profile of the tunnel barrier in the direct tunnelling regime [41] . Regarding the scalability of FTJs, Pantel et al. [43] reported large TER (OFF/ON=300) with Co/PbZr 0.2 Ti 0.8 O 3 / La 0.7 Sr 0.3 MnO 3 triangular-shaped tunnel junctions with an effective diameter of 220 nm. OFF/ON ratios of 10,000 were shown in Co/BiFeO 3 /Ca 0.96 Ce 0.04 MnO 3 tunnel junctions with diameters of 180 nm ( Fig. 3a ) [7] . Gao et al. [38] showed indications of TER with I versus V DC (OFF/ON >100 at large voltage) on 20-nm-wide Ag/BaTiO 3 /SrRuO 3 junctions. Further investigations are needed to ensure switchable polarization for junctions with diameters <100 nm. 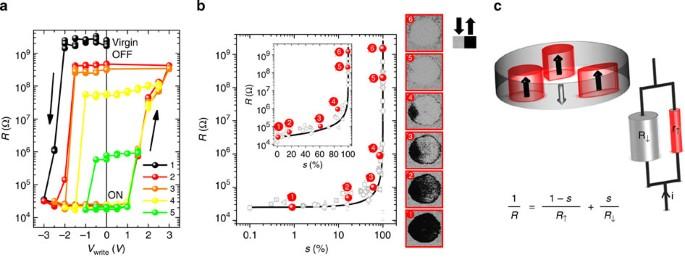Figure 3: Non-uniform ferroelectric domain configurations and memristive behaviour. Pt/Co/BiFeO3(4.5 nm)/Ca0.96Ce0.04MnO3junctions with diameters of 180 nm. (a) These BiFeO3-based junctions exhibit OFF/ON ratio of 10,000 after applying 100 ns voltage pulses. Intermediate resistance states are stabilized by decreasing the maximum voltage pulses amplitude. (b) Correlation between various resistance states from ON to OFF (and OFF to ON) and the corresponding fraction of down domains (s) deduced from PFM images from 10 different junctions of the same size. PFM images for six different resistance states (red dots) of one of the junctions are displayed. The black line is a calculation from the parallel resistance model sketched inc, with the expression of the resistance as a function ofsand the resistance of each (down or up) domain. (Adapted, with permission, from ref.7, copyright 2013 American Chemical Society.) Figure 3: Non-uniform ferroelectric domain configurations and memristive behaviour. Pt/Co/BiFeO 3 (4.5 nm)/Ca 0.96 Ce 0.04 MnO 3 junctions with diameters of 180 nm. ( a ) These BiFeO 3 -based junctions exhibit OFF/ON ratio of 10,000 after applying 100 ns voltage pulses. Intermediate resistance states are stabilized by decreasing the maximum voltage pulses amplitude. ( b ) Correlation between various resistance states from ON to OFF (and OFF to ON) and the corresponding fraction of down domains (s) deduced from PFM images from 10 different junctions of the same size. PFM images for six different resistance states (red dots) of one of the junctions are displayed. The black line is a calculation from the parallel resistance model sketched in c , with the expression of the resistance as a function of s and the resistance of each (down or up) domain. (Adapted, with permission, from ref. 7 , copyright 2013 American Chemical Society.) Full size image In addition to the use of FTJs as digital binary memory with two resistance states corresponding to two orientations of the ferroelectric polarization, non-uniform ferroelectric domain configurations can be exploited in order to build multistate digital memories [46] or memristors [47] . Hysteresis variations of the remnant resistance versus write voltage pulses of 300-nm-wide Co/BaTiO 3 /La 0.7 Sr 0.3 MnO 3 junctions show that intermediate resistance states between the ON and OFF states can be stabilized depending on the amplitude history of write voltage pulses [39] . Using PFM imaging through the top electrode of these junctions, Chanthbouala et al. [39] mapped the evolution of ferroelectric domains for various intermediate resistance states from ON to OFF and back to ON. The progressive resistance evolution between ON and OFF in Co/BaTiO 3 /La 0.7 Sr 0.3 MnO 3 junctions is correlated to the switching of the ferroelectric polarization from up (towards Co) to down (towards La 0.7 Sr 0.3 MnO 3 ) through the progressive nucleation in several zones with limited propagation. A simple model of parallel conduction through up and down ferroelectric domains ( Fig. 3c ) allows the correlation between resistance and ferroelectric domain population. Yamada et al. [7] reported giant TER effects (OFF/ON=10,000) with 180-nm-wide Co/BiFeO 3 /Ca 0.96 Ce 0.04 MnO 3 tunnel junctions ( Fig. 3a ). The films were grown on YAlO 3 substrates that stabilizes the polymorphic T-phase of BiFeO 3 with giant tetragonality for which a very large ferroelectric polarization is expected [48] , [49] , [50] . The resistance variation of the junctions was correlated to the switching of polarization through images of ferroelectric domains ( Fig. 3b ). In the virgin state, the polarization is pointing down (towards Ca 0.96 Ce 0.04 MnO 3 , bright-phase signal) and the resistance is high, whereas in the ON state the polarization is pointing up (towards Co, dark-phase contrast; Fig. 3a,b ). Intermediate resistance states consist of a mixed population of up and down ferroelectric domains; the evolution of ferroelectric domains with the resistance is reversible. Once again, parallel domain conduction ( Fig. 3c ) was validated with the comparison of ferroelectric domain images and resistance measurements of multiple devices (black line in Fig. 3b ). The correlation between the resistance of BaTiO 3 (ref. 39 ) and BiFeO 3 (ref. 7 ) tunnel junctions in various intermediate states and the parallel resistance model suggests a negligible (if any) contribution from the ferroelectric domain walls in the tunnel resistance [51] , [52] . The agreement between ferroelectric domain configurations and resistance indicates that the dynamics of ferroelectric domains in such nanostructures can be easily probed by tunnel resistance measurements as a function of voltage pulses. The resistance of the Co/BaTiO 3 /La 0.7 Sr 0.3 MnO 3 junctions can be progressively increased (or decreased) by applying cumulative 20 ns voltage pulses of the same intermediate positive (or negative) amplitude [39] . Hence, this memristive behaviour emulates the typical plasticity of synapses and could be implemented in neuromorphic architectures [53] . As the tunnelling current is highly sensitive to the electronic properties of the ferroelectric/electrode interfaces in FTJs, the electrode material can be specifically chosen to exhibit large modifications of its electronic properties with the electric field provided by the ferroelectric. Wen et al. [8] demonstrated very large OFF/ON ratios >10 4 with BaTiO 3 -based tunnel junctions ( Fig. 4b ). They chose Nb:SrTiO 3 crystal substrates (with Nb varying from 0.1 to 1%) as bottom semiconducting electrodes and large (30 μm) Pt pads as top electrodes. The similarity between coercive voltages of ferroelectric switching, detected via PFM loops through the 30-nm top electrodes ( Fig. 4c ), and those of resistance switching ( Fig. 4b ) confirmed the ferroelectric origin of the effect. The large resistance contrast was interpreted by the carrier depletion/accumulation in the semiconductor by the field effect created by the polarization of the 3.4-nm-thick BaTiO 3 tunnel barrier. When the polarization of BaTiO 3 is pointing away from the semiconductor, electron carriers are depleted that adds an additional Schottky barrier to the tunnel barrier and drastically increases the resistance in the OFF state ( Fig. 4a ). This concept was validated by the dependence of the OFF/ON ratio with the dopant concentration in the semiconductor: the lower the Nb concentration, the higher the Schottky barrier and the higher the OFF state ( Fig. 4d ). 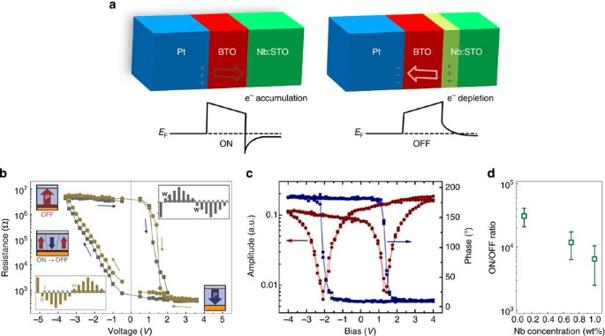Figure 4: One semiconductor electrode boosts the TER. (a) Sketch of the electron band diagram of a ferroelectric tunnel junction consisting in a BaTiO3(BTO) ultrathin film sandwiched between a Pt metallic electrode and a Nb:SrTiO3(STO) semiconducting electrode. When the ferroelectric polarization points to the right, electrons from the semiconductor are accumulated to screen the positive charges of polarization. This bends down the conduction band and lowers the barrier height of BTO; the device is in the ON state. When the polarization is pointing to the left, electrons carriers are depleted from the semiconductor resulting in an additional Schottky barrier at the BTO/Nb:STO interface. This widens the tunnelling barrier and drastically increases the OFF state of the device (adapted from ref.96). (b) Resistance hysteresis loops of Pt/BTO/Nb:STO ferroelectric tunnel junctions at room temperature. The loop composed of dark squares (green circles) is measured using the pulse train shown schematically in the top-right (bottom-left ) inset. The device is preset to the ON (OFF) state by a positive (negative) 3.6 V pulse. The testing pulse train is composed of write pulses following a triangular profile between +3.6 and −3.6 V, and read pulses of +0.1 V following each write pulse. The corresponding domain evolution is shown schematically in the bottom-right, top-left and middle-left insets for the ON, OFF and intermediate states, respectively. (c) PFM phase and amplitude hysteresis loops of the Pt/BTO/Nb:STO ferroelectric tunnel junctions. (d) ON/OFF ratio read at +0.1 V as a function of Nb doping concentration in Nb:STO. The data points show averages over 20 devices for each Nb concentration. ((b–d) Adapted from ref.8.) Figure 4: One semiconductor electrode boosts the TER. ( a ) Sketch of the electron band diagram of a ferroelectric tunnel junction consisting in a BaTiO 3 (BTO) ultrathin film sandwiched between a Pt metallic electrode and a Nb:SrTiO 3 (STO) semiconducting electrode. When the ferroelectric polarization points to the right, electrons from the semiconductor are accumulated to screen the positive charges of polarization. This bends down the conduction band and lowers the barrier height of BTO; the device is in the ON state. When the polarization is pointing to the left, electrons carriers are depleted from the semiconductor resulting in an additional Schottky barrier at the BTO/Nb:STO interface. This widens the tunnelling barrier and drastically increases the OFF state of the device (adapted from ref. 96 ). ( b ) Resistance hysteresis loops of Pt/BTO/Nb:STO ferroelectric tunnel junctions at room temperature. The loop composed of dark squares (green circles) is measured using the pulse train shown schematically in the top-right (bottom-left ) inset. The device is preset to the ON (OFF) state by a positive (negative) 3.6 V pulse. The testing pulse train is composed of write pulses following a triangular profile between +3.6 and −3.6 V, and read pulses of +0.1 V following each write pulse. The corresponding domain evolution is shown schematically in the bottom-right, top-left and middle-left insets for the ON, OFF and intermediate states, respectively. ( c ) PFM phase and amplitude hysteresis loops of the Pt/BTO/Nb:STO ferroelectric tunnel junctions. ( d ) ON/OFF ratio read at +0.1 V as a function of Nb doping concentration in Nb:STO. The data points show averages over 20 devices for each Nb concentration. (( b – d ) Adapted from ref. 8 .) Full size image Another interesting way to increase the OFF/ON ratio is to induce an interfacial metal/insulator phase transition by the electric field created by the ferroelectric polarization. Yin et al. [42] grew an ultrathin layer of La 0.5 Ca 0.5 MnO 3 in all-oxide epitaxial La 0.7 Sr 0.3 MnO 3 /La 0.5 Ca 0.5 MnO 3 (0.8 nm)/BaTiO 3 /La 0.7 Sr 0.3 MnO 3 tunnel junctions. The manganite material La x Ca 1− x MnO 3 with x =0.5 is intentionally chosen at the frontier between a ferromagnetic metallic phase (for x <0.5) and an antiferromagnetic insulating phase (for x >0.5) at low temperature [54] . The concept is that the adjacent ferroelectric polarization of BaTiO 3 will either deplete or accumulate carriers (holes) in the ultrathin layer of La 0.5 Ca 0.5 MnO 3 , which is equivalent to a shift in the phase diagram of the manganite to x <0.5 or x >0.5, respectively ( Fig. 5a ). Hence, switching the ferroelectric polarization could induce a phase transition in the ultrathin La 0.5 Ca 0.5 MnO 3 . For reference La 0.7 Sr 0.3 MnO 3 /BaTiO 3 /La 0.7 Sr 0.3 MnO 3 junctions with a 3-nm-thick BaTiO 3 layer, a low TER of 0.3 (or OFF/ON ratio of 1.3) is measured at 40 K. This value is compatible with an asymmetry of the interface terminations that can induce a small TER [16] ( Fig. 5c ). For La 0.7 Sr 0.3 MnO 3 /La 0.5 Ca 0.5 MnO 3 (0.8 nm)/BaTiO 3 /La 0.7 Sr 0.3 MnO 3 tunnel junctions measured in the same conditions ( V DC =10 mV after applying increasing/decreasing voltage pulses of 20 ms), the TER strongly increases by two orders of magnitude (50 at 40 K and up to 100 at 5 K; Fig. 5d ). The high and low resistances when the polarization points away and towards La 0.5 Ca 0.5 MnO 3 , respectively, validate the concept of a metal/insulator phase transition in La 0.5 Ca 0.5 MnO 3 triggered by the ferroelectric polarization. The modulation of the tunnel resistance induced by the phase transition when switching the ferroelectric polarization was validated by ab initio calculations with matching TER amplitudes ( Fig. 5b ) [55] . 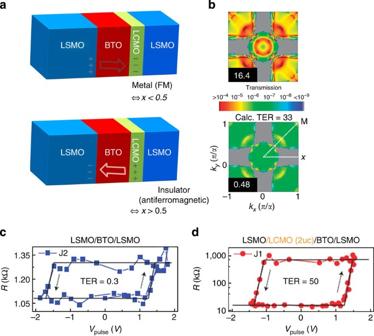Figure 5: Enhanced TER with electric field induced phase transition. (a) Sketch of the heterostructure with the screening charge accumulation in the La0.7Sr0.3MnO3(LSMO) and La0.5Ca0.5MnO3(LCMO) electrodes for opposite ferroelectric polarization orientations in the BaTiO3(BTO) layer. When the polarization points to the right, holes are depleted, which makes LCMO metallic and ferromagnetic (FM). When it points to the left, holes are accumulated, and LCMO becomes insulating and antiferromagnetic. (b) Results of density functional calculations with kk-resolved distribution of the tunnelling transmission in the two-dimensional Brillouin zone for the two corresponding states depicted ina. The integrated total conductance G per in-plane cell is given in the lower-left corner of each plot (in units of 10−6e2h−1). Note that the colour scale is logarithmic and the grey areas correspond to zero transmission. The resulting TER is calculated to be 33. (c,d) Resistance memory loops measured atVDC=10 mV as a function of voltage pulses (20 ms) at 40 K for (c) LSMO/BTO (3 nm)/LSMO and (d) LSMO/LCMO (0.8 nm)/BTO (3 nm)/LSMO junctions. (Adapted from ref.42.) Figure 5: Enhanced TER with electric field induced phase transition. ( a ) Sketch of the heterostructure with the screening charge accumulation in the La 0.7 Sr 0.3 MnO 3 (LSMO) and La 0.5 Ca 0.5 MnO 3 (LCMO) electrodes for opposite ferroelectric polarization orientations in the BaTiO 3 (BTO) layer. When the polarization points to the right, holes are depleted, which makes LCMO metallic and ferromagnetic (FM). When it points to the left, holes are accumulated, and LCMO becomes insulating and antiferromagnetic. ( b ) Results of density functional calculations with kk-resolved distribution of the tunnelling transmission in the two-dimensional Brillouin zone for the two corresponding states depicted in a . The integrated total conductance G per in-plane cell is given in the lower-left corner of each plot (in units of 10 −6 e 2 h −1 ). Note that the colour scale is logarithmic and the grey areas correspond to zero transmission. The resulting TER is calculated to be 33. ( c , d ) Resistance memory loops measured at V DC =10 mV as a function of voltage pulses (20 ms) at 40 K for ( c ) LSMO/BTO (3 nm)/LSMO and ( d ) LSMO/LCMO (0.8 nm)/BTO (3 nm)/LSMO junctions. (Adapted from ref. 42 .) Full size image Very recently, Jiang et al. [56] investigated interfacial phase transitions in PbZr 0.2 Ti 0.8 O 3 (10 nm)/La 1− x Sr x MnO 3 (5 nm) heterostructures with a C-AFM tip as top electrode. They exploited the rich phase diagram of La 1− x Sr x MnO 3 , and observed a change in the sign of the TER by changing the electrode composition between x =0.20 and x =0.50. These results were explained by polarization-induced phase transitions: when the ferroelectric polarization of PbZr 0.2 Ti 0.8 O 3 points towards La 1− x Sr x MnO 3 , it induces hole depletion resulting in a metal to insulator or insulator to metal transitions, for x =0.20 or x =0.50, respectively. These results emphasize how FTJs can be used as powerful tools to induce and probe interfacial phase transitions. Coupling ferroelectrics with magnetic materials may enable a control of magnetism by an electric field. Interfacial magnetoelectric effects have aroused large interest over the past few years [57] . Significant changes of the magnetic properties at the ferroelectric/metal interface can appear due to screening effects [58] , [59] , [60] , [61] , changes of the interface bonding [62] , [63] , [64] , [65] and changes of the interfacial magnetocrystalline anisotropy [66] . The reversible electric field induced by the ferroelectric is predicted to induce interesting features, such as (i) a modification of the magnetization of an adjacent ferromagnet [58] , [62] ; (ii) the stabilization of ferromagnetism in a paramagnetic metal [59] ; or (iii) ferromagnetic/antiferromagnetic phase transitions [61] . In spintronics, a key building block is the magnetic tunnel junction where two ferromagnetic electrodes sandwich an ultrathin layer of dielectric [67] . In these devices, the tunnel resistance has two distinct states corresponding to the antiparallel or parallel configurations of the magnetic electrodes (which are controllable by a magnetic field). This effect, called tunnel magnetoresistance (TMR), is based on spin-dependent electron tunnelling that is extremely sensitive to the spin-dependent electronic properties of the ferromagnet/dielectric interface. Hence, measurements of TMR can be used to probe interfacial changes of the magnetic properties. The interplay between ferroelectricity and ferromagnetism can be investigated through transport measurements in artificial multiferroic tunnel junctions, in which a ferroelectric tunnel barrier is sandwiched between two ferromagnetic electrodes [68] . The two ferroic order parameters (ferromagnetism and ferroelectricity) give rise to four distinct resistance states ( Fig. 6a ) owing to the combined TMR and TER effects. Interface magnetoelectric coupling between the ferroelectric and the ferromagnetic can be probed by measuring the modulation of the spin-dependent tunnelling current (through the TMR). 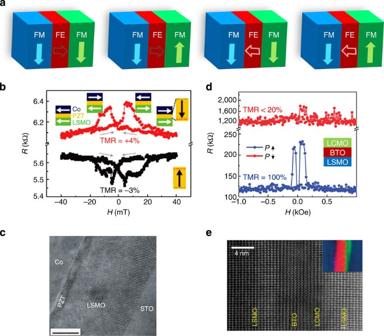Figure 6: Ferroelectric (FE) control of spin-polarization. (a) Sketch of artificial multiferroic tunnel junctions consisting of two ferromagnetic (FM) electrodes separated by a FE tunnel barrier. The FE polarization (open arrow) is controlled by an electric field, whereas the configuration of the electrodes magnetizations (solid arrows) are controlled by a magnetic field, giving rise to four non-equivalent resistance states. (b) Resistance (R) versus magnetic field (H) curves measured atVDC=10 mV and 50 K in the as-grown state of a Co/PZT (3.2 nm)/LSMO junction (black squares) and after polarization switching with a +3-V applied electrical bias (red circles). The polarization states of the barrier as well as magnetization directions in each magnetic layer are schematically shown for each non-volatile state. (c) High-resolution transmission electron microscopy image of the same heterostructure. ((b,c) Adapted from ref.73.) (d)RversusHfor a LSMO/LCMO (0.8 nm)/BTO (3 nm)/LSMO tunnel junction in the high- (top) and low- (bottom) resistance states atVDC=10 mV and 80 K. (e) Cross-section annular dark-field scanning transmission electron microscopy image of the same heterostructure. ((d,e) Adapted from ref.42.) LSMO, PZT, STO, LCMO and BTO stand for La0.7Sr0.3MnO3, PbZr0.2Ti0.8O3, SrTiO3, La0.5Ca0.5MnO3and BaTiO3, respectively. Figure 6: Ferroelectric (FE) control of spin-polarization. ( a ) Sketch of artificial multiferroic tunnel junctions consisting of two ferromagnetic (FM) electrodes separated by a FE tunnel barrier. The FE polarization (open arrow) is controlled by an electric field, whereas the configuration of the electrodes magnetizations (solid arrows) are controlled by a magnetic field, giving rise to four non-equivalent resistance states. ( b ) Resistance ( R ) versus magnetic field ( H ) curves measured at V DC =10 mV and 50 K in the as-grown state of a Co/PZT (3.2 nm)/LSMO junction (black squares) and after polarization switching with a +3-V applied electrical bias (red circles). The polarization states of the barrier as well as magnetization directions in each magnetic layer are schematically shown for each non-volatile state. ( c ) High-resolution transmission electron microscopy image of the same heterostructure. (( b , c ) Adapted from ref. 73 .) ( d ) R versus H for a LSMO/LCMO (0.8 nm)/BTO (3 nm)/LSMO tunnel junction in the high- (top) and low- (bottom) resistance states at V DC =10 mV and 80 K. ( e ) Cross-section annular dark-field scanning transmission electron microscopy image of the same heterostructure. (( d , e ) Adapted from ref. 42 .) LSMO, PZT, STO, LCMO and BTO stand for La 0.7 Sr 0.3 MnO 3 , PbZr 0.2 Ti 0.8 O 3 , SrTiO 3 , La 0.5 Ca 0.5 MnO 3 and BaTiO 3 , respectively. Full size image Gajek et al. [69] were the first to demonstrate the existence of a four resistance state memory using a multiferroic (ferroelectric and ferromagnetic) tunnel barrier of La 0.1 Bi 0.9 MnO 3 sandwiched between La 0.7 Sr 0.3 MnO 3 and Au electrodes . Artificial multiferroic tunnel junctions are easier to realize because multiferroics that are both ferromagnetic and ferroelectric are rare, and it is difficult to decouple their magnetization when used as a tunnel barrier from that of the ferromagnetic electrode. Ab initio calculations performed on Fe/BaTiO 3 interfaces showed a large interface magnetoelectric coupling resulting from a modification of the ferromagnet/ferroelectric interface bonding upon switching of the ferroelectric polarization [62] . Sizeable modifications of the Fe- and Ti-induced magnetic moments at the Fe/BaTiO 3 interface have been calculated by several groups [62] , [64] , [65] . In order to probe this interfacial magnetoelectric coupling, Fe/BaTiO 3 (1.2 nm)/La 0.7 Sr 0.3 MnO 3 nanoscale tunnel junctions were fabricated. X-ray resonant magnetic scattering on these heterostructures revealed that the induced magnetic moment on the Ti is coupled to the Fe electrode [70] , which is in agreement with ab initio predictions [62] , [64] , [71] . The tunnel junctions exhibited negative TMR at 4 K, indicating that the Fe/BaTiO 3 interface tunnel spin-polarization is negative, as predicted by ab initio calculations [62] , [64] , [71] . The ferroelectric polarization of BaTiO 3 was switched with voltage pulses of +1/−1 V and 1 s duration, and the TMR was subsequently measured while sweeping the magnetic field and collecting the current at V DC =−50 mV in the different ferroelectric states. Large changes of the negative TMR were observed depending on the orientation of the ferroelectric polarization: the TMR is large (small) when the ferroelectric polarization points towards Fe (La 0.7 Sr 0.3 MnO 3 ) (ref. 72 ). The variation of the TMR with the ferroelectric polarization can reach 450%. Hence, the ferroelectric tunnel barrier provides a way to efficiently control the spin-polarization of the tunnel current, locally, in a non-volatile manner and potentially with a low energy [72] . Pantel et al. [73] showed that, with large area Co/PbZr 0.2 Ti 0.8 O 3 (3.2 nm)/La 0.7 Sr 0.3 MnO 3 tunnel junctions ( Fig. 6c ), it is even possible to reverse the sign of the TMR by switching the ferroelectric polarization. They performed magnetotransport measurements at V DC =10 mV and 50 K, and observed a change of the TMR from −3 to +4% when the ferroelectric polarization was pointing to the Co or the La 0.7 Sr 0.3 MnO 3 , respectively ( Fig. 6b ). Although the TMR is not large, its relative variation with the ferroelectric polarization reaches −230%. Thus, the orientation of the ferroelectric polarization of the PbZr 0.2 Ti 0.8 O 3 tunnel barrier controls the sign of the current spin-polarization, providing potential for electrically controlled spintronic devices [73] . In the experiments by Yin et al. [42] , the use of the interfacial La 0.5 Ca 0.5 MnO 3 layer was shown to induce large modifications of the TMR in La 0.7 Sr 0.3 MnO 3 /La 0.5 Ca 0.5 MnO 3 (0.8 nm)/BaTiO 3 /La 0.7 Sr 0.3 MnO 3 junctions ( Fig. 6e ) while switching the ferroelectric polarization of the barrier. As illustrated in Fig. 5a , the polarization-induced metal/insulator phase transition in La 0.5 Ca 0.5 MnO 3 is accompanied by a ferromagnetic/antiferromagnetic transition. Hence, at 80K, the TMR is ~100% (close to zero) when the ferroelectric polarization points towards (away from) La 0.5 Ca 0.5 MnO 3 corresponding to its ferromagnetic (antiferromagnetic) state ( Fig. 6d ). An interfacial magnetic phase transition driven by the ferroelectric polarization of the tunnel barrier is thus an efficient way to control the spin-polarization of the tunnel current: the variation of the TMR with the ferroelectric polarization orientation reaches 500% in this specific case. All the above-mentioned experiments of ferroelectric control of spin-polarization ( Table 2 ) use at least one ferromagnetic electrode of La 0.7 Sr 0.3 MnO 3 , thereby limiting the experiments to operation below room temperature [74] . Moreover, thermally activated inelastic tunnelling processes through defects in the ferroelectric tunnel barrier can limit both TER and TMR at higher temperature [42] , [44] , [75] . Nevertheless, Yin et al. showed a four-state memory at room temperature with La 0.7 Sr 0.3 MnO 3 /Ba 0.95 Sr 0.05 TiO 3 (3.5 nm)/La 0.7 Sr 0.3 MnO 3 tunnel junctions, albeit with extremely small contrasts of resistance (<1%) and no apparent variations of the spin-dependent signal with the ferroelectric polarization orientation [76] ( Table 2 ). Systems with solely transition metals or their alloys as bottom and top electrodes should be investigated to look for efficient ferroelectric control of spin-polarization at room temperature. Table 2 Survey of experimental reports with artificial multiferroic tunnel junctions. Full size table Solid-state FTJs investigated within the last couple of years have shown promising properties as non-volatile resistive memory elements, including large OFF/ON ratios [7] , [8] , reproducibility [7] , [37] , high speed [37] , [39] and potentially low operation energy [37] . Besides their use as binary memories, FTJs also have great potential as memristive devices for possible implementations as artificial synapses in neuromorphic architectures [39] . These ferroelectric memristors will be interconnected to artificial neural networks to demonstrate unsupervised learning with bio-inspired rules such as spike-timing-dependent plasticity [53] . Despite this fast recent progress, the field of FTJs is, however, still in its genesis, and there is high potential for improvement both from technological and fundamental perspectives. Technologically, specific attention should be paid to the endurance of FTJs that is currently limited to the order of 10 6 (refs 7 , 8 , 37 , 77 ). FeRAMs based on thick ferroelectric films were shown to have very high endurance (>10 14 cycles) [78] ; the right combination of ferroelectric/electrode materials must be found to reach this goal in FTJs. Defects such as oxygen vacancies in the tunnel barrier are critical for endurance; they can be investigated by advanced PFM imaging experiments [79] or temperature- and voltage-dependent transport measurements. The retention of these nanodevices will also be critical. Importantly, the scalability of FTJs is not limited by its readout process, in contrast to the case of classical FeRAMs. FTJs with dimensions of the order of 200 nm have been demonstrated [7] , [36] , [43] , and there are some preliminary results with devices <100 nm (refs 30 , 37 , 38 ). Investigations on nanoscale tunnel junctions are required to evaluate the limit of scalability of the devices and assess their potential as non-volatile memories and as memristors in massively parallel architectures [80] . Also decisive for the applicative development of FTJs will be their compatibility with CMOS electronics. FTJs based on epitaxial-strained oxide ferroelectrics require specific substrates and high processing temperatures, although atomic layer deposition may allow growth below 300 °C (ref. 81 ). Organic ferroelectrics [82] are an interesting alternative as they can be deposited at or near room temperature. Ferroelectricity was demonstrated in ultrathin films of organics such as PVDF-TrFE (poly(vinylidene fluoride) with trifluoroethylene) over a decade ago [21] , [83] , but to date, experimental reports of TER with organic ferroelectric tunnel barriers remain scarce. In 2005, Qu et al. [84] observed conductivity modulation associated with polarization reversal in two monolayer-thick PVDF-TrFE films through scanning tunnelling microscopy experiments. Recently, Kusuma and Lee [85] fabricated junctions with six monolayer-thick VDF (vinylidene fluoride) ferroelectric tunnel barriers and reported an OFF/ON ratio of 10 with an endurance of 10 4 with these organic FTJs. First principles calculations of PVDF tunnel barriers embedded between ferromagnetic electrodes predict large modulations of the TMR with the ferroelectric polarization, and suggest exciting interplay between the organic/ferromagnetic interface hybridization and the spintronic response of the device, thereby opening a route to highly flexible multifunctional devices [86] , [87] . From a fundamental point of view, the interplay between ferroelectric/metal interface properties and the tunnelling current flowing through FTJs is still not well understood. The role of ferroelectricity in the resistive switching process is now established, with the correlation of the tunnel resistance with non-uniform configurations of ferroelectric domains observed within the devices by PFM [7] , [39] , [43] . However, some influence of electrochemical phenomena correlated with ferroelectric polarization switching cannot be completely excluded [40] . Alongside with a b initio calculations [42] , [55] , investigations of the actual metal/ferroelectric interfaces with spectroscopic techniques, such as X-ray photoemission spectroscopy [41] and advanced transmission electron microscopy-based techniques [88] , [89] , will bring further insights on the understanding of TER. To control the preferential orientation and switchability of ferroelectric films, as well as the switching processes and polarization dynamics, interface engineering [88] , [90] at the atomic level will be necessary. In addition, with judiciously chosen materials, electric field effect-mediated changes of the electronic properties at the electrode/barrier interfaces can strongly enhance the TER signal [8] , [42] . The functional properties of strongly correlated materials are highly dependent on the carrier concentration and may be manipulated with electric field [91] . Mott insulators [92] such as rare-earth nickelates could be used as electrodes to electrically induce a metal–insulator transition by the ferroelectric tunnel barrier with possibly large TER. The ferroelectric control of superconductivity [93] and ferromagnetism [60] in FTJs is also of great interest. Beyond charge-based electronics, there is an avenue for the non-volatile electrical control of spintronic devices integrating these ferroelectric tunnel barriers. Ferroelectric field effect could also modulate the magnetic properties of paramagnetic metals that are close to the Stoner criterion for itinerant ferromagnetism [59] . Such a paramagnetic/ferromagnetic phase transition may be detected by performing electrically controlled spin-dependent transport in artificial multiferroic tunnel junctions. The sign of spin-currents may be manipulated by coupling heavy metals with ferroelectrics and electrically controlling the Rashba spin splitting [94] . More generally, ferroelectrics have strong potential to bring low-power, non-volatile, voltage-based control of spin-currents in the nascent field of spin-orbitronics [95] . How to cite this article: Garcia, V. and Bibes, M. Ferroelectric tunnel junctions for information storage and processing. Nat. Commun. 5:4289 doi: 10.1038/ncomms5289 (2014).